Direct electrochemical oxidation of alcohols with hydrogen evolution in continuous-flow reactor Alcohol oxidation reactions are widely used for the preparation of aldehydes and ketones. The electrolysis of alcohols to carbonyl compounds have been underutilized owing to low efficiency. Herein, we report an electrochemical oxidation of various alcohols in a continuous-flow reactor without external oxidants, base or mediators. The robust electrochemical oxidation is performed for a variety of alcohols with good functional group tolerance, high efficiency and atom economy, whereas mechanistic studies support the benzylic radical intermediate formation and hydrogen evolution. The electrochemical oxidation proves viable on diols with excellent levels of selectivity for the benzylic position. Aldehydes or ketones are not only essential functionalities of various biologically active compounds, but also important reagents in modern organic synthesis [1] , [2] . In fact, the high frequently used of alcohol oxidations to carbonyl compounds leading to a ranking of 3rd of strongly prefer better reagents for pharmaceutical manufacturers [3] . So, developing oxidation of alcohols under environmentally benign and economic conditions is highly demanded [4] , [5] , [6] , [7] for pharmaceutical and chemical industries. Stoichiometric oxidants such as chromium, manganese, and ruthenium salts [8] , [9] , [10] , [11] , [12] , [13] , [14] , [15] are relatively not environmental friendly (Fig. 1a ). Molecular oxygen, air, or hydrogen peroxide in combination with appropriate transition metal catalysts (Cu, Ru, Pd, Au, Fe, V, or Ir) [16] , [17] , [18] , [19] , [20] , [21] , [22] represent superior alternatives according to the principles of green and sustainable chemistry. However, the oxidation remains challenging for a broad group of alcohols. In contrast, oxidant-free alcohol oxidation with hydrogen evolution is apparently an ideal process to reach the higher atom economy (Fig. 1b ). This concept has been achieved with transition metal catalysis [23] , [24] , [25] , [26] , [27] , [28] , [29] , [30] , which normally involves expensive transition metals, sophisticated ligands, and generally requires high reaction temperatures. On the other hand, alcohol oxidation with hydrogen release via photocatalysis [31] , [32] or electrocatalysis [33] , [34] , [35] , [36] , [37] , [38] , [39] , [40] have the merit of running reactions under mild conditions. Fig. 1 Alcohol oxidation conditions. a Alcohols oxidation with oxidant. b Alcohols oxidation with dehydrogenation. c Alcohol oxidation under continuous-flow set-up Full size image Direct electrolysis of alcohols to carbonyl compounds is an idealized goal, which produces only hydrogen without product contamination. The direct electro-oxidation of alcohol can be tracked back to the pioneering work of Lund and Mayeda et al. [41] , [42] , [43] using undivided electrolysis cells. However, prior attempts gave only the desired aldehydes or ketones in low selectivity and efficiency. We envisioned that electrolysis in a continuous-flow set-up would be a sustainable method to replace stoichiometric oxidants and improve both energy efficiency and productivity. Large surface-to-volume ratio, enhanced mass transfer, operation at quasi-isothermal condition, and lower resistances are the advantages of using flow electrochemistry set-up, which often make it superior than batch mode [44] , [45] , [46] . In addition, the electrode surface can be regenerated efficiently to avoid low conductivity for the transformations with gas evolution. Furthermore, flow cells are easy to scale up and employed in industry [47] , [48] , [49] . Recently, electrochemical flow cells have been successfully used in a variety of organic transformations [50] , [51] , [52] , [53] , [54] , [55] , [56] , [57] , [58] , [59] , [60] , [61] , [62] , [63] , [64] . Herein, we report the direct electrolysis of alcohols to afford the aldehydes or ketones with high efficiency without any mediators or catalysts under neutral conditions by using a flow reactor (Fig. 1c and Supplementary Fig. 1 ). 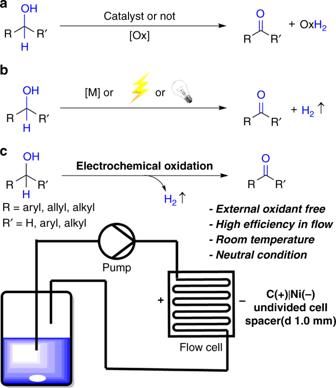Fig. 1 Alcohol oxidation conditions.aAlcohols oxidation with oxidant.bAlcohols oxidation with dehydrogenation.cAlcohol oxidation under continuous-flow set-up Investigation of reaction conditions Our studies commenced with benzyl alcohol ( 1aa ), which was subjected to a batch condition in an undivided cell (Table 1 , entry 1), yielding 37% of benzaldehyde ( 2aa ) at 100 mA constant current electrolysis for 1 h (Supplementary Fig. 2 ). In order to improve the solubility of the starting material, CH 3 CN and water (1:1) were used as solvents in the continuous-flow set-up, and benzaldehyde ( 2aa ) was isolated in 93% yield under the same current (10 mA, 10 h, Table 1 , entry 2). Encouraged by these results, we investigated the magnitude of current from 10 mA to 1000 mA (entries 2–8). When 50 mA was applied for the oxidation, 92% of benzaldehyde was isolated in 2 h (Table 1 , entry 3). Among a set of studies, 800 mA enabled effective oxidation up to 99% yield in 10 min (Table 1 , entry 7). However, when the current was increased to 1000 mA, 2aa was provided in lower yield (81%, entry 8). The flow rate was another parameter, which was evaluated at the current of 800 mA. Accordingly, 0.10 mL s −1 was the optimum flow rate (Table 1 , entries 9–11). Then the reaction conditions of 800 mA, 10 min and 0.10 mL s −1 were employed for the further researches. Table 1 Optimization of electrochemical oxidation of benzyl alcohol 1aa Full size table At the flow rate of 0.10 mL s −1 , the solution passed through the flow cell multiple times by using peristaltic pump. We think that it would be possible to achieve full conversion by employing large current and small flow rate. By using this strategy, the 2 mmol benzyl alcohol in 30 mL mixed solvent could be quantitatively transformed to benzyaldehyde at 800 mA and 0.02 mL s −1 in 25 min (Fig. 2a and Supplementary Fig. 3 ). Furthermore, the reaction scale can be extended to 100.0 mmol at the same current and the flow rate still in quantitative yield (Fig. 2b and Supplementary Fig. 4 ). These results illustrated the potential applicability of this method. Fig. 2 Slow flow rate of electrochemical oxidation of benzyl alcohol 1aa . a The amount of 1aa is 2.0 mmol. b The amount of 1aa is 100.0 mmol Full size image Substrate scope With the optimized reaction conditions in hand, we next explored various benzylic and allylic alcohols 1ab-1ap (2.0 mmol) under galvanostatic conditions (Fig. 3 ). Electron-rich benzylic alcohols with ortho- , meta- , and para -substitution could be converted to the corresponding aldehydes 2ab-2ah in nearly quantitative yields (96–99%) without over oxidation. Halogenated benzylic alcohols could be oxidized to afford the corresponding aldehydes 2ai-2ak in excellent yield (98–99%), which could be further functionalized. Owing to weak C–I bond, 10 mA cell current had to be adapted and 4-iodo benzaldehyde ( 2al ) was obtained in moderate yield (60%). Moreover, electron-deficient benzylic alcohols gave less satisfactory results. For example, compound 2am was obtained in only 35% yield. On the other hand, 1-naphthyl methanol ( 1an ) was converted to the corresponding aldehyde 2an in 88% yield. The flow conditions could also be applied to thiophene derivative 1ao to afford aldehyde 2ao in 76% yield without significant side product formation. Additionally, we explored the possibility of electrolysis of allylic alcohol 1ap , thus obtaining the corresponding unsaturated aldehyde 2ap in 64% yield. Fig. 3 Substrate scopes of electrochemical oxidation of primary alcohols. Reaction conditions: carbon paper (93 × 93 × 0.2 mm) anode (contact area 1.6 cm 2 ), Ni plate (93 × 93 × 0.3 mm) cathode (contact area 1.6 cm 2 ), constant current = 800 mA, flow rate = 0.10 mL s −1 , 10 min, 1a (2.0 mmol), n Bu 4 NBF 4 (0.20 mmol), CH 3 CN/H 2 O (1:1, 30 mL), N 2 , room temperature, flow cell (2.49 F mol −1 ), isolated yield. a 10 mA, 10 h. b 10 mA, 20 h Full size image The reaction conditions were subsequently employed to oxidize a range of secondary alcohols (Fig. 4 ). Excellent results were observed for oxidation of alcohols 1ba - 1bf to the corresponding ketones 2ba-2bf in 83–97% yield. There was no significant difference in the reactivity of primary and secondary alcohols in the continuous-flow reactor. The oxidation of heterocyclic alcohol 1bg proceeded smoothly under 10 mA cell current condition to afford ketone 2bg in 70% yield. Oxidation of allylic alcohols 1bh − 1bi afforded the desired ketones in 50–75% yield. However, aliphatic alcohol was not oxidized smoothly under electrochemical oxidation condition and gave 2bj in 25% yield. Fig. 4 Substrate scopes of electrochemical oxidation of secondary alcohols. Reaction conditions: carbon paper (93 × 93 × 0.2 mm) anode (contact area 1.6 cm 2 ), Ni plate (93 × 93 × 0.3 mm) cathode (contact area 1.6 cm 2 ), constant current = 800 mA, flow rate = 0.10 mL s −1 , 10 min, 1b (2.0 mmol), n Bu 4 NBF 4 (0.20 mmol), CH 3 CN/H 2 O (1:1, 30 mL), N 2 , room temperature, flow cell (2.49 F mol −1 ), isolated yield. a 10 mA, 20 h. b 10 mA, 10 h. c 1be : benzoin used as starting material Full size image This observation led us to explore the selective oxidation of diols 3 and 5 as shown in Fig. 5 . For both substrates, benzylic hydroxyl groups were oxidized selectively in the presence of aliphatic primary or secondary hydroxyl groups to afford hydroxyl ketones 4 and 6 in 78% and 85% yields, respectively. This oxidation could be complementary to Swern oxidation, which is selective for primary or less steric hindered alcohols [65] , [66] , [67] . Fig. 5 Selective oxidation of benzylic alcohols in the presence of aliphatic alcohols. a Selective oxidation of 1-phenylbutane-1,3-diol. b Selective oxidation of 1-phenylbutane-1,4-diol Full size image The continuous-flow electrolysis was further extended to pharmaceutical relevant substrates (Fig. 6 ). Rosuvastatin precursor 1aq [68] could be oxidized to the corresponding aldehyde in 76% yield within only 10 min, which presented the potential application prospect of this protocol. Fluorenol ( 1bk ) [69] was oxidized to the corresponding ketones in good yields (86%). Fig. 6 Electrochemical oxidation of biologically relevant substrates. a Electrochemical oxidation of Rosuvastatin precursor. b Electrochemical oxidation of 9 H -fluoren-9-ol Full size image The possibility of using water as solvent was also estimated. However, benzaldehyde was obtained in only 82% yield due to the poor solubility of alcohols in water. Thus, the surfactant was employed and we noted that the ionic surfactant could also be the supporting electrolyte. By using this strategy, benzaldehyde could be prepared in quantitative yield in water (Fig. 7 ). Six primary alcohols in Fig. 3 and four secondary alcohols in Fig. 4 have been chosen to re-evaluate the yields in the presence of surfactant in pure water. In general, aqueous conditions provided the desired products in comparable yields with our standard conditions, which showed that the combination of water and surfactant would be a good choice for this protocol. Fig. 7 Substrate scopes of electrochemical oxidation of alcohols in water. Reaction conditions: carbon paper (93 × 93 × 0.2 mm) anode (contact area 1.6 cm 2 ), Ni plate (93 × 93 × 0.3 mm) cathode (contact area 1.6 cm 2 ), constant current = 800 mA, flow rate = 0.10 mL s −1 , 10 min, 1 (2.0 mmol), N,N,N -trimethylhexadecan-1-ammonium sulfate (0.10 mmol), H 2 O (15 mL), N 2 , room temperature, flow cell (2.49 F mol −1 ), isolated yield. a LiClO 4 instead of N,N,N -trimethylhexadecan-1-ammonium sulfate. b 10 mA, 20 h. c 10 mA, 10 h Full size image Since the oxidation of alcohol in the anode means the loss of electron, the existence of radical intermediate is highly probable. To gain insight into the reaction mechanism, electron paramagnetic resonance (EPR) experiments were performed by adding the radical spin trapping agent DMPO (5, 5-dimethyl-1-pyrroline N-oxide). No radical signal was detected in the absence of 1aa (Fig. 8a , blank line). When DMPO was added to the reaction under constant current conditions, a radical signal ( g = 2.0069, A N = 14.82, A H = 21.42) was identified (Fig. 8a , red line). According to the fitting result, this radical signal came from benzyl radical captured by DMPO. Fig. 8 Mechanistic studies experiments. a EPR results of benzyl alcohol oxidation. b D 2 O and H 2 18 O labeling experiments. c Kinetic profiles under different concentrations of 1aa . d Kinetic profiles under different current Full size image No deuterium or 18 O was incorporated into benzaldehyde when H 2 O was substituted with D 2 O or H 2 18 O in the reaction system (Fig. 8b and Supplementary Figs. 5 and 6 ). This result indicated that water did not react with the intermediate under the reaction conditions. This was in accordance with no over oxidation to benzoic acid was observed even when benzaldehyde was used as starting material for this electrolysis (Supplementary Fig. 8 ). In addition, no over oxidation of the aldehyde products may also benefit from the fact that no extra base was added in our reaction system. The influence of the concentration, current, and flow rate to the electrochemical oxidation of benzyl alcohol have been evaluated as shown in Fig. 8 . Reaction rate increased with the increasing of the concentration of benzyl alcohol (Fig. 8c ). It was the same that large current meant high reaction rate (Fig. 8d ). The reaction rate kept unchanged when the flow rate was larger than 0.10 mL s −1 (Supplementary Fig. 7 ). These results suggested that the electrochemical oxidation was likely to be the rate-limiting step during electrolysis. On the basis of our mechanistic studies and literature reports [41] , [42] , [43] , a possible mechanism for the oxidation of alcohols to carbonyl functionality is depicted in Fig. 9 . The oxidation of benzyl alcohol was initiated by anodic oxidation to afford intermediate B . The consequent deprotonation of the radical cation B resulted in the formation of benzylic radical C , which has been detected by EPR. The following fast single-electron oxidation and deprotonation of D produce the desired benzaldehyde ( 2aa ). Lower efficiency of oxidation with electron deficient benzylic alcohols could be explained by considering that electron withdrawing groups destabilized intermediates. In the meantime, water underwent cathodic reduction to generate hydroxide accompanied by releasing hydrogen [70] . The in situ formed hydroxide acted as base to trap the protons. For the whole reaction, no external oxidant was needed, which is in accordance with the idea of green chemistry. Fig. 9 Proposed mechanism of benzyl alcohol electrochemical oxidation. A tentative reaction mechanism involves anodic oxidation of benzyl alcohol to afford intermediate B , deprotonation, single electron oxidation and deprotonation to form the desired benzaldehyde ( 2aa ). Water underwent cathodic reduction to generate hydroxide accompanied by releasing hydrogen Full size image In summary, a direct electrochemical oxidation of alcohols to the corresponding carbonyl compounds has been accomplished efficiently by the continuous-flow reactor just using carbon anode. Reactions were performed without external oxidant, mediator or additive and no over oxidation was observed, which make this method an ideal transformation from alcohols to aldehydes or ketones. Even water can be used as solvent in the presence of surfactant. The reaction conditions have been applied for selective oxidation and biologically relevant substrates. The reaction can be adjusted conveniently from milligram to gram scale based on demand by using the flow set-up. Further research to broaden the substrate scope of alcohol oxidation will be reported in due course. General procedures for the electrolysis in acetonitrile and water In an oven-dried schlenck tube (100 mL) equipped with a stir bar, alcohol 1a (2.0 mmol), n Bu 4 NBF 4 (65.9 mg, 0.2 mmol) and CH 3 CN/H 2 O (1:1, 30 mL) were added. The flow cell was equipped with carbon paper (9.3 cm × 9.3 cm × 0.2 mm) as the anode (contact area 1.6 cm 2 ) and nickel plate (9.3 cm × 9.3 cm × 0.3 mm) as the cathode (contact area 1.6 cm 2 ). In order to preclude the possibility that air was involved in the oxidation of alcohol, we flushed the whole system with nitrogen before the direct electrolysis. The reaction mixture was pumped into the electrochemical reactor at the flow rate of 0.10 mL s −1 (Supplementary Fig. 1 ). Method A: A constant current of 800 mA was employed during the electrolysis under room temperature for 10 min. (Method B: A constant current of 10 mA was employed during the electrolysis under room temperature for 10 h. Method C: A constant current of 10 mA was employed during the electrolysis under room temperature for 20 h.) When the reaction was finished, the reaction mixture was washed with water and extracted with dichloromethane (10 mL x 3). 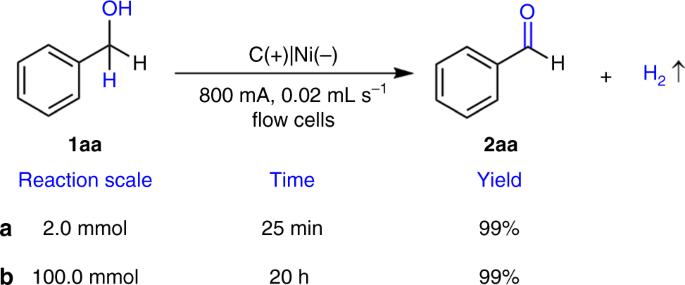Fig. 2 Slow flow rate of electrochemical oxidation of benzyl alcohol1aa.aThe amount of1aais 2.0 mmol.bThe amount of1aais 100.0 mmol The organic layers were combined, dried over Na 2 SO 4 , and concentrated. The pure product was obtained by flash column chromatography on silica gel using petroleum ether and ethyl acetate as the eluent. General procedures for the electrolysis in water with surfactant Method D: In an oven-dried schlenck tube (100 mL) equipped with a stir bar, alcohol 1a (2.0 mmol), N,N,N -trimethylhexadecan-1-ammonium sulfate (69.6 mg, 0.10 mmol) and H 2 O (15 mL) were added. The flow cell was equipped with carbon paper (9.3 cm × 9.3 cm × 0.2 mm) as the anode (contact area 1.6 cm 2 ) and nickel plate (9.3 cm × 9.3 cm × 0.3 mm) as the cathode (contact area 1.6 cm 2 ). In order to preclude the possibility that air was involved in the oxidation of alcohol, we flushed the whole system with nitrogen before the direct electrolysis. The reaction mixture was pumped into the electrochemical reactor in a flow rate of 0.10 mL s −1 (Supplementary Fig. 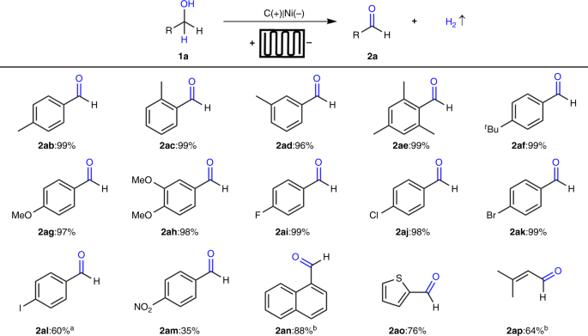Fig. 3 Substrate scopes of electrochemical oxidation of primary alcohols. Reaction conditions: carbon paper (93 × 93 × 0.2 mm) anode (contact area 1.6 cm2), Ni plate (93 × 93 × 0.3 mm) cathode (contact area 1.6 cm2), constant current = 800 mA, flow rate = 0.10 mL s−1, 10 min,1a(2.0 mmol),nBu4NBF4(0.20 mmol), CH3CN/H2O (1:1, 30 mL), N2, room temperature, flow cell (2.49 F mol−1), isolated yield.a10 mA, 10 h.b10 mA, 20 h 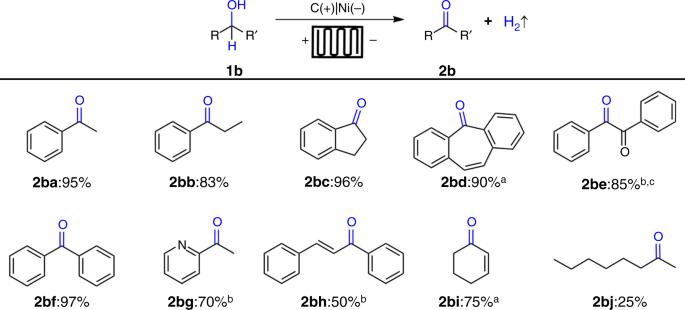Fig. 4 Substrate scopes of electrochemical oxidation of secondary alcohols. Reaction conditions: carbon paper (93 × 93 × 0.2 mm) anode (contact area 1.6 cm2), Ni plate (93 × 93 × 0.3 mm) cathode (contact area 1.6 cm2), constant current = 800 mA, flow rate = 0.10 mL s−1, 10 min,1b(2.0 mmol),nBu4NBF4(0.20 mmol), CH3CN/H2O (1:1, 30 mL), N2, room temperature, flow cell (2.49 F mol−1), isolated yield.a10 mA, 20 h.b10 mA, 10 h.c1be: benzoin used as starting material 1 ). A constant current of 800 mA was employed during the electrolysis under room temperature for 10 min. When the reaction was finished, the reaction mixture was washed with water and extracted with dichloromethane (10 mL x 3). 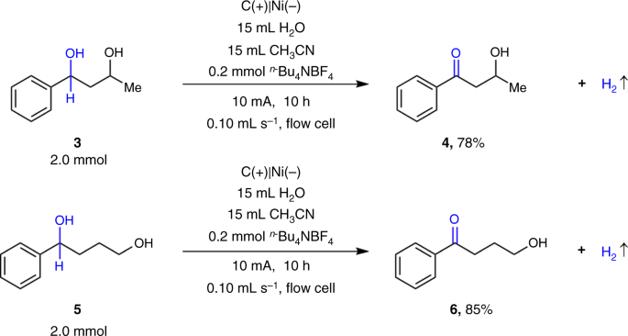Fig. 5 Selective oxidation of benzylic alcohols in the presence of aliphatic alcohols.aSelective oxidation of 1-phenylbutane-1,3-diol.bSelective oxidation of 1-phenylbutane-1,4-diol The organic layers were combined, dried over Na 2 SO 4 , and concentrated. 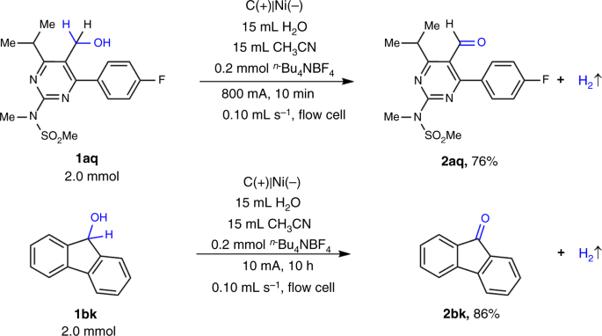Fig. 6 Electrochemical oxidation of biologically relevant substrates.aElectrochemical oxidation of Rosuvastatin precursor.bElectrochemical oxidation of 9H-fluoren-9-ol 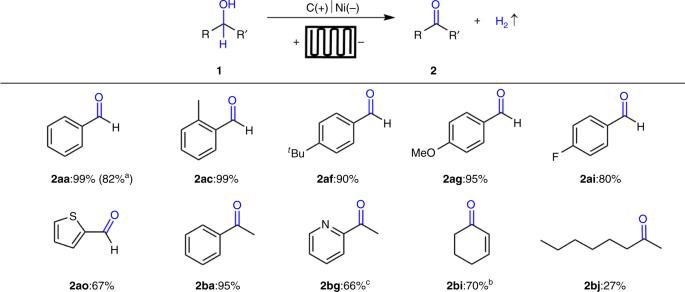Fig. 7 Substrate scopes of electrochemical oxidation of alcohols in water. Reaction conditions: carbon paper (93 × 93 × 0.2 mm) anode (contact area 1.6 cm2), Ni plate (93 × 93 × 0.3 mm) cathode (contact area 1.6 cm2), constant current = 800 mA, flow rate = 0.10 mL s−1, 10 min,1(2.0 mmol),N,N,N-trimethylhexadecan-1-ammonium sulfate (0.10 mmol), H2O (15 mL), N2, room temperature, flow cell (2.49 F mol−1), isolated yield.aLiClO4instead ofN,N,N-trimethylhexadecan-1-ammonium sulfate.b10 mA, 20 h.c10 mA, 10 h 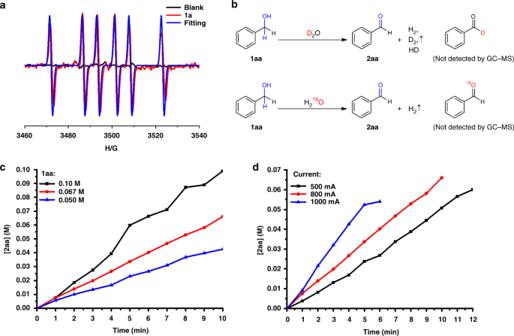Fig. 8 Mechanistic studies experiments.aEPR results of benzyl alcohol oxidation.bD2O and H218O labeling experiments.cKinetic profiles under different concentrations of1aa.dKinetic profiles under different current 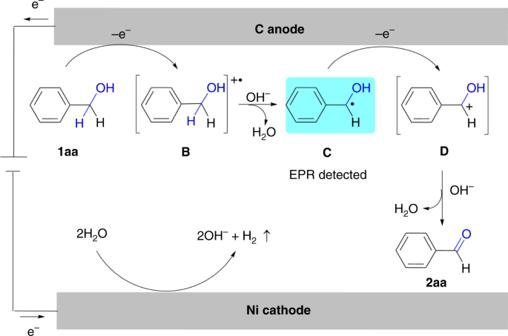Fig. 9 Proposed mechanism of benzyl alcohol electrochemical oxidation. A tentative reaction mechanism involves anodic oxidation of benzyl alcohol to afford intermediateB, deprotonation, single electron oxidation and deprotonation to form the desired benzaldehyde (2aa). Water underwent cathodic reduction to generate hydroxide accompanied by releasing hydrogen The pure product was obtained by flash column chromatography on silica gel using petroleum ether and ethyl acetate as the eluent.